Observation of higher stiffness in nanopolycrystal diamond than monocrystal diamond Diamond is the stiffest known material. Here we report that nanopolycrystal diamond synthesized by direct-conversion method from graphite is stiffer than natural and synthesized monocrystal diamonds. This observation departs from the usual thinking that nanocrystalline materials are softer than their monocrystals because of a large volume fraction of soft grain-boundary region. The direct conversion causes the nondiffusional phase transformation to cubic diamond, producing many twins inside diamond grains. We give an ab initio- calculation twinned model that confirms the stiffening. We find that shorter interplane bonds along [111] are significantly strengthened near the twinned region, from which the superstiff structure originates. Our discovery provides a novel step forward in the search for superstiff materials. Polycrystalline materials often show different mechanical properties compared with corresponding monocrystals. Solids possess two especially important mechanical properties. First is the strength, which relates closely with hardness. Grain boundaries affect the macroscopic strength. They increase or decrease the strength, depending on the grain size, known as Hall–Petch or reverse Hall–Petch strengthening. Second is the elastic stiffness, which reflects resistance to elastic deformation of the lattice structure. Unlike strength, the elastic stiffness of a polycrystal has always been reported to be lower than that of the corresponding monocrystal. This trend becomes large as the grain size decreases because of increased intercrystalline region. Korn et al . [1] reported that Young’s moduli of nanocrystalline CaF 2 , Pd and Mg were 38, 88 and 39 GPa, respectively, which are 34%, 65% and 87%, respectively, of those predicted from corresponding monocrystals by the Hill averaging method [2] . There are many similar reports: Nieman et al . [3] reported decrease in Young’s modulus in nanocrystalline Pd and Cu by 50–85% and 65–72%, respectively. For nanocrystalline Fe [4] and Al [5] , the moduli are 65–85% and 20–60% of the monocrystal, respectively. For Cu thin films, the longitudinal-wave modulus is about 80% of the predicted value [6] ; in addition, one could cite many more examples. The stiffness inherently reflects interatomic potential and is proportional to the second derivative of the energy with respect to strain. Considering lattice anharmonicity, such a softening is attributed to the larger free volume at the grain boundaries [7] . Also, the macroscopic stiffness decreases considerably when the material contains noncohesive intergrain bonds, because displacement increases when a softer region is stressed [8] , [9] . Thus, low stiffness in nanopolycrystals is well established. Diamond is the hardest and stiffest material. However, Irifune et al . [10] found an even harder material: nanopolycrystalline diamond (NPD) with an average grain size about several tens of nanometres. They made their nanopolycrystal diamond from graphite under high pressure (>12 GPa) and high temperature (>2300 °C), without metallic binders. Its Knoop hardness is about 130 GPa at room temperature, exceeding that of high-purity monocrystal diamond (60–120 GPa) [11] , [12] . This superhardness was attributed to the blocking of dislocation movement by grain boundaries and lamellar structures [12] , [13] , being analogous to Hall–Petch strengthening. On the other hand, the elastic stiffness in a nanopolycrystal is expected to be lower because of the grain-boundary regions. Here we found that the NPD is significantly stiffer than the monocrystal diamond. This superstiffening remained undiscovered, because it has been difficult to measure the stiffness of diamond accurately with conventional ultrasonic methods because obtainable specimens are small and diamonds exhibit extremely high sound velocity. We use Brillouin-oscillation signals [14] using picosecond ultrasound for measuring the longitudinal-wave modulus C near the specimen surface [15] . It obviously exceeds the monocrystal diamond value. We proposed twinned superlattice structure models to explain this superstiff behaviour and confirmed their stiffness enhancement using ab initio calculations. Furthermore, we found that the shorter interplane bonds at and near the twinned region were largely strengthened, making the entire microstructure stiffer. Specimens We fabricated 15 direct-conversion-sintering NPD specimens (DC-NPDs) (specimen nos 1–14 and 43), 13 monocrystal diamond specimens (specimen nos 15–27) using the temperature-gradient method [16] , [17] , epitaxial chemical-vapour-deposition (CVD) diamonds on monocrystal diamond substrate using a microwave-plasma CVD method (nos 28–31) and polycrystalline diamond specimens by a microwave-plasma CVD method without (CVD-micropolycrystalline diamond (CVD-MPD), nos 32–35) and with (CVD-NPD, nos 36–42) nitrogen gas. Adding nitrogen gas significantly decreases the grain size through formation of nuclei [18] , [19] . 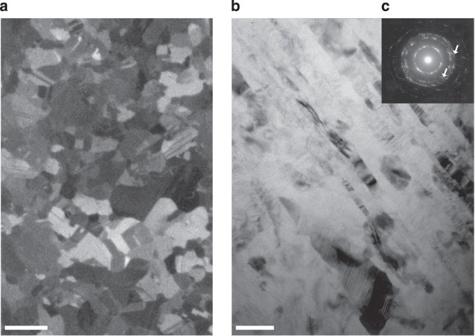Figure 1: Twinned microstructures. (a) A scanning-electron-microscopy image, indicating twinned structures inside most grains. Scale bar, 200 nm. (b) A transmission electron microscopy image, showing fine grains, and (c) its diffraction pattern, where streaks appear (indicated by arrows), indicating twinned structures. Scale bar, 50 nm (b). Figure 1 shows a typical microstructure of a DC-NPD specimen observed by scanning electron microscopy and transmission electron microscopy, showing fine grains and many twins inside the grains. Using X-ray diffraction, we confirmed that the DC-NPD specimens consist of equiaxially oriented cubic diamond grains without significant texture, involving no other phases such as graphite and hexagonal diamond ( Supplementary Fig. S1 ). Figure 1: Twinned microstructures. ( a ) A scanning-electron-microscopy image, indicating twinned structures inside most grains. Scale bar, 200 nm. ( b ) A transmission electron microscopy image, showing fine grains, and ( c ) its diffraction pattern, where streaks appear (indicated by arrows), indicating twinned structures. Scale bar, 50 nm ( b ). 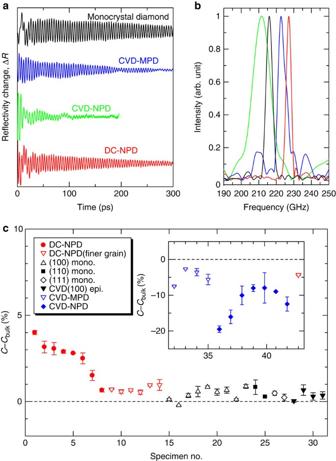Figure 2: Elastic constant measurement. (a) Brillouin-oscillation waveforms for various diamond specimens, and (b) corresponding Fourier spectra. (c) Longitudinal-wave elastic constant of all the specimens.Cbulkdenotes the elastic constant calculated by Miglioriet al.20values. Error bars represent s.d. among independent measurements at 5–10 different points on each specimen. CVD(100) epi., CVD diamond epitaxially grown on (100) monocrystal diamond. Full size image Elastic constants Figure 2a and b shows typical Brillouin-oscillation waveforms and corresponding Fourier spectra of four kinds of specimens, respectively. The Brillouin-oscillation frequency of a DC-NPD specimen is clearly higher than those of CVD-MPD and CVD-NPD diamonds, which were synthesized by conventional methods, indicating higher stiffness of DC-NPD. Figure 2: Elastic constant measurement. ( a ) Brillouin-oscillation waveforms for various diamond specimens, and ( b ) corresponding Fourier spectra. ( c ) Longitudinal-wave elastic constant of all the specimens. C bulk denotes the elastic constant calculated by Migliori et al . [20] values. Error bars represent s.d. among independent measurements at 5–10 different points on each specimen. CVD(100) epi., CVD diamond epitaxially grown on (100) monocrystal diamond. Full size image Figure 2c plots the elastic constants of all the specimens, where the vertical axis expresses the difference from the reported value of cubic diamond. (Several reports appear for the elastic constants of cubic diamond, and we adopted the values by Migliori et al . [20] , because they used the most accurate method among others: resonance ultrasound spectroscopy. Their values at room temperature are C 11 =1078.6 GPa, C 12 =126.6 GPa and C 44 =577.6 GPa, and the averaged longitudinal-wave stiffness C =1156.7 GPa.) The monocrystal diamonds and epitaxial CVD diamonds show slightly higher stiffness than the previous monocrystal value. This is attributed to higher purity of the diamonds synthesized in this study: the temperature-gradient method allows us to synthesize diamonds with impurities less than several tens p.p.m. [16] , [17] , and the CVD method with high-purity gases also yields high-purity diamonds. The stiffness of CVD-MPD is lower than the monocrystal value by 3–8%, and that of CVD-NPD is markedly lower by 10–20%. This observation is well acceptable because of larger volume fraction of the grain-boundary region. Noncohesive intergrain bonds also explain their softer behaviour. However, DC-NPDs show clearly higher stiffness than the monocrystal diamond (except for no. 43), despite their much finer grains than CVD-MPDs and CVD-NPDs. The increment value of DC-NPD reaches 3% compared with the monocrystals (specimen nos 15–31). This is a surprising observation because no other materials can be stiffened by their polycrystallization: DC-NPD is the only material that stiffens during nanopolycrystallization and is stiffer than monocrystal diamond. Considering that the degree of the stiffness enhancement is less remarkable for finer-grain DC-NPDs, we expect that there must be a mechanism that makes the innergrain structure stiffer. We observed twinned structures inside grains entirely in DC-NPD specimens ( Fig. 1 ). Because of the direct conversion from graphite, nearly nondiffusional phase transition occurs, producing twins. Actually, twinned structures were observed in highly plastically deformed diamonds [21] . Twin structures are known to increase the strength and hardness significantly through obstruction of dislocation movements [22] , [23] . However, there is no report on elastic stiffening enhancement caused by twins because they were recognized only as lattice defects, which usually cause elastic softening. To study the influence of twinned structure on the stiffness in diamond, we propose superlattice-like twinned structures with various twin-boundary volume fractions, where twin boundaries exist periodically along <111> in cubic diamond ( Fig. 3 ), and their elastic constants were calculated using ab initio calculation. Because the twin-boundary structure along [111] of cubic diamond is identical to the stacking structure of hexagonal diamond (lonsdaleite), we also calculated the elastic constants of hexagonal diamond as the extreme case of the maximum volume fraction of twinned region. We used QUANTUM ESPRESSO code [24] , which is based on a plane-wave pseudopotential approach to the density functional theory [25] . The generalized gradient approximation (GGA) method was used to treat the exchange-correlation function. The energy cutoff value of the plane-wave expansion for the wave function was 60 Ry, and that of the charge density was 600 Ry. The k -point mesh for the calculations was 8 × 8 × 8 Monkhorst-Pack scheme [26] . The calculation took three steps. First, we performed optimization of the proposed structures, which yielded atomic forces <10 −6 Ry Å −1 and an energy variation <10 −8 Ry, indicating sufficiently optimized structures. Second, we determined the five independent elastic constants of the proposed structures using the relationships between applied strain and energy increase of the system as shown in Supplementary Fig. S2 . (Note that the proposed structures are transversely isotropic.) Third, we calculated the averaged-overdirection elastic constants using Hill’s averaging method [2] . 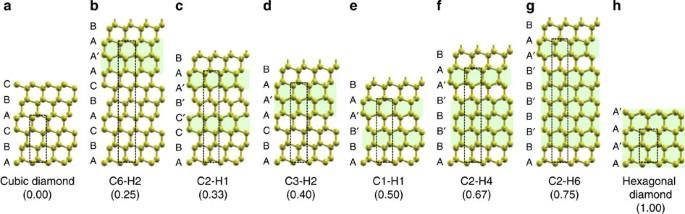Figure 3: Superlattice-like twinned structure models. The (111) cubic diamond (a) and hexagonal diamond (h) show ABCABC... and AA′AA′... stacking, respectively, where A′ denotes π-rotated A plane. Six twinned structures (b–g) are proposed in this study. Cm-Hnindicates that the unit structure consists ofmcubic-diamond-like interplane bonds andnhexagonal-diamond-like interplane bonds. Light-green regions correspond to the twinned region. The structureccorresponds to a purely twinned cubic-diamond structure, and other models are anomalous twinned structures, which are recognized as polytypes. Note that many other such structures can be constructed. Figure 3: Superlattice-like twinned structure models. The (111) cubic diamond ( a ) and hexagonal diamond ( h ) show ABCABC... and AA′AA′... stacking, respectively, where A′ denotes π-rotated A plane. Six twinned structures ( b – g ) are proposed in this study. C m -H n indicates that the unit structure consists of m cubic-diamond-like interplane bonds and n hexagonal-diamond-like interplane bonds. Light-green regions correspond to the twinned region. The structure c corresponds to a purely twinned cubic-diamond structure, and other models are anomalous twinned structures, which are recognized as polytypes. Note that many other such structures can be constructed. 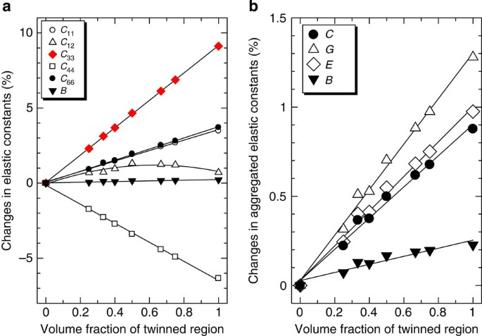Figure 4: Elastic constants of twinned structures. (a) Five independent elastic constants of the twinned structures. (b) Bulk modulusB, shear modulusG, Young’s modulusEand longitudinal-wave modulusCof aggregates of the twinned structures. Full size image Figure 4a shows the independent elastic constants of the twinned structures as a function of the volume fraction of twinned region (light-green regions in Fig. 3 ). The interplane distances of the (111) cubic-diamond structure agreed with measurements within 0.02% ( Supplementary Table S1 ), confirming the reliability of the optimization procedure. As the volume fraction increases, the out-of-plane longitudinal elastic constant C 33 increases significantly. Figure 4b shows the aggregated (polycrystalline) elastic constants, clearly showing that principal elastic constants increase as twinning increases. Thus, twins in cubic diamond stiffen the structure, and this model can explain the stiffness increase in DC-NPD. We also performed similar elastic-constant calculations for the twinning structures of Si. The results are shown in Supplementary Fig. S3 . The elastic constants of the twin-superlattice structures showed similar trends with those of twinned diamonds ( Supplementary Fig. S3a ). However, the aggregated elastic constants decrease as the increase of the twinned region ( Supplementary Fig. S3b ). One of the remarkable properties of diamond is its very high shear modulus. The ratio of the shear modulus to the bulk modulus is about 1.2 for cubic diamond, whereas that of Si is 0.67. In Fig. 4a , C 33 increases by 9% and C 44 decreases by 0.6% from cubic to hexagonal phases. On the other hand, for Si, C 33 increases by again 9%, but C 44 decreases by 14% as shown in Supplementary Fig. S3a . Therefore, the twinned region significantly decreases the out-of-plane shear modulus in Si, resulting in the decreases in the principal polycrystalline elastic constants. Thus, twins in Si make the structure softer, and this is expected because twins are recognized as defects. Diamond keeps its high shear modulus even when twinning is introduced. Therefore, the twin-stiffening mechanism is a unique characteristic of cubic diamond. Figure 4: Elastic constants of twinned structures. ( a ) Five independent elastic constants of the twinned structures. ( b ) Bulk modulus B , shear modulus G , Young’s modulus E and longitudinal-wave modulus C of aggregates of the twinned structures. Full size image Further investigation was performed to identify the stiffening mechanism. As shown in Fig. 4a , the stiffness enhancement along [111] ( C 33 ) is remarkable in the twin-diamond structures, and this contributes highly to the increase in the aggregated stiffness. We therefore calculated the local effective spring constant by computing energy increment by applying local deformation along [111] to the interatomic bonds in the twinned structures in Fig. 3 . We here focus on two representative interplane bonds, as shown in Fig. 5 , named short (S) bonds and long (L) bonds. For example, there are five kinds of S bonds and four kinds of L bonds in the C6-H2 model, and there are four kinds of S-bonds and five kinds of L-bonds in C2-H6 model. The results are shown in Fig. 6 for the two models. We found that S-bond spring constants in the twinned region are markedly increased; they increase towards the S-bond value in hexagonal diamond as the volume fraction increases. On the other hand, the L-bond spring constant is comparable or slightly lower in the twinned regions. Therefore, strengthened S bonds at and near twinned regions cause the stiffened structure of DC-NPD. 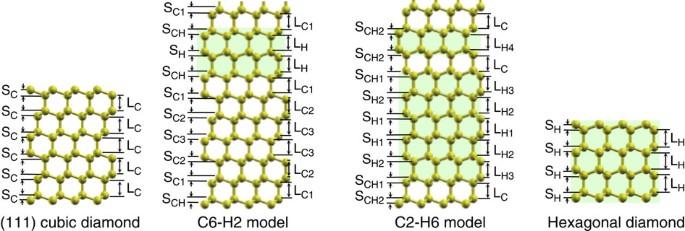Figure 5: Two representative interplane bonds. SHand LHdenote short and long interplane bonds inside twinned region, respectively. SCHdenotes the short bond at the interface. SCand LCare short and long bonds in the cubic-diamond-structure region, respectively. Figure 5: Two representative interplane bonds. S H and L H denote short and long interplane bonds inside twinned region, respectively. S CH denotes the short bond at the interface. S C and L C are short and long bonds in the cubic-diamond-structure region, respectively. 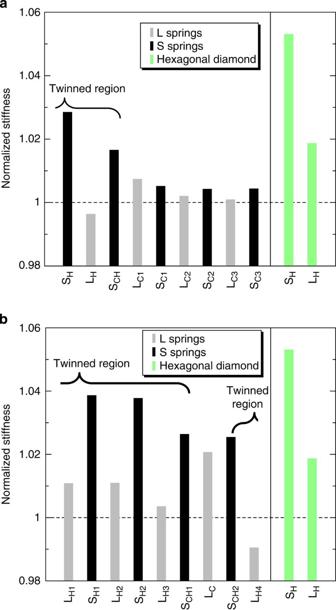Figure 6: Local-spring-constant distributions. (a) C6-H2 model and (b) C2-H6 model. The S- and L-bond spring constants are normalized by those of cubic diamond (SC=1.056 × 1022N m−3and LC=0.684 × 1022N m−3). The spring constants in hexagonal diamond are also shown with green bars for comparison. Full size image Figure 6: Local-spring-constant distributions. ( a ) C6-H2 model and ( b ) C2-H6 model. The S- and L-bond spring constants are normalized by those of cubic diamond (S C =1.056 × 10 22 N m −3 and L C =0.684 × 10 22 N m −3 ). The spring constants in hexagonal diamond are also shown with green bars for comparison. Full size image The predicted elastic-constant increment (<1%) is smaller than the measurement (<3%). This will be attributed to the fact that a few per cent discrepancy between ab initio -calculation stiffness and measured stiffness is acceptable as shown in Supplementary Table S2 . Another possible reason is the nonrelaxed structures of DC-NCD specimens. Because of the nondiffusional direct conversion from graphite, lattice structures will be highly strained, which depart from fully relaxed structures used in the theoretical calculation. Furthermore, such an extreme synthesizing condition could cause unidentified polytypes. Our twin model is a subset of diamond polytypes. Wen et al . [27] calculated the elastic constants of 10 diamond polytypes, and we calculated the aggregated longitudinal-wave modulus C using their calculation results ( Supplementary Fig. S4 ). There is, however, no polytype to achieve the 3% stiffness increase; the stiffness increment is comparable with our twin model, whereas the correlation between the hexagonality and the stiffness increase is poorer. Some polytypes decrease the stiffness. Therefore, the twinned-structure model is currently promising for the stiffness-enhancement mechanism among various polytype structures. However, an undiscovered polytype, which yields a much higher C value, might exist. In summary, we showed that NPD is stiffer than monocrystal diamond, the stiffest known material, using picosecond ultrasound spectroscopy and that this stiffening mechanism can be explained by twins inside the cubic diamond grains using an ab initio calculation. Twinned diamond seems to be the only material whose stiffness exceeds diamond. The S-bond strength inside the twinned region is significantly enhanced, which causes ultrastiff structure in cubic diamond. The principal elastic constants of hexagonal diamond are theoretically higher than those of cubic diamond ( Fig. 4 ), and hexagonal diamond is expected to be a candidate superstiff material. However, it is unstable under atmospheric pressure [28] . Thus, only twins in cubic diamond can achieve the superstiff behaviour. Specimen fabrication We fabricated the DC-NPD specimens under a pressure of 12–16 GPa at 1,900–2,300 °C from high-purity (>99.99%) graphite compacts of various grain sizes. We changed the resultant grain size by changing synthesis conditions and grain size of the source material. Grain sizes of DC-NPD specimens were 50–100 nm for nos 1–8, 30–50 nm for nos 9–14 and 10–30 nm for no. 43. For comparison, we synthesized monocrystal diamonds with (100) (nos 15–23), (110) (nos 24 and 25) and (111) (nos 26 and 27) faces under 5.5 GPa at 1,350 °C. Also, we fabricated epitaxial CVD diamonds on (100) monocrystal diamond substrate using a microwave-plasma CVD method, with a source gas composed of methane and hydrogen gases. Furthermore, polycrystalline diamond specimens (CVD-MPD and CVD-NPD) were synthesized by a microwave-plasma CVD method. Grain size of CVD-MPD was 1–5 μm, and that of CVD-NPD was 100–500 nm. Picosecond ultrasound spectroscopy The picosecond-ultrasound method was first proposed by Thomsen et al . [29] , [30] It uses ultrashort pump light pulses for generating ultrahigh-frequency elastic wave in the direction perpendicular to the specimen surface principally through thermal expansion of the surface region of material, and probe light pulses for detecting coherent phonons in the material through the photoelastic effect. Because the frequency range of the generated elastic-wave pulse reaches terahertz order, the picosecond-ultrasound method has been a powerful tool for studying mechanical properties of thin films and nanostructure materials. Usually, a single Ti-sapphire pulse laser was used in this method, where a single light pulse was divided into pump and probe pulses. With this measurement setup, however, it was difficult to change pulse width of pump and probe lights independently. Also, this setup requires many optical elements, through which the pulse width enlarges. We need narrower pulse width (shorter pulse) in the pump light for generating higher-frequency elastic waves, but wider pulse width (hopefully monochromatic light) in the probe light for detecting the Brillouin-oscillation frequency with higher accuracy. Thus, we used two femtosecond pulse lasers with different pulse widths of 100 fs for pumping and 200 fs for probing. Our optics is shown in Supplementary Fig. S5 . The 100-fs pulse-width Ti-S laser (master) was for pumping, and the 200-fs pulse-width laser (slave) was for probing. They were synchronized within about 50 fs by adjusting the cavity length of the slave-pulse laser with a piezoelectric stage by comparing the timing of the slave-pulse laser with that of the master-pulse laser. The pump light pulse entered a TiO 2 acousto-optic crystal for amplitude modulation, and the first-order diffracted light was perpendicularly focused on the specimen surface through the objective lens. The probe light pulse was frequency-doubled and also focused perpendicularly on the specimen surface. The half-bandwidths of pump (800 nm) and probe (400 nm) lights at the specimen surface were about 10 and 1 nm, respectively, realizing short and long pulses for pumping and probing, respectively. A 10-nm aluminium thin film was deposited on each specimen surface for generating the acoustic pulse via thermal expansion. The backward diffraction of the probe light pulse caused by the acoustic pulse is enhanced when the wavelength of the probe light inside the specimen equals the twofold wavelength of the acoustic wave. This Bragg’s condition gives the sound velocity of the acoustic wave V as V = fλ /(2 n ), where f , λ and n denote the Brillouin-oscillation frequency, wavelength of the probe light in vacuum and refractive index of the specimen, respectively. n was obtained by an ellipsometry method with accuracy >0.1% as shown below. Mass density ρ was determined with accuracy of 0.3% by a gas-expansion pycnometer for specimen volume and a microbalance for specimen mass. The longitudinal-wave modulus C was obtained by C = ρV 2 . The possible maximum error in the measured elastic constant is, therefore, 0.4%, which is significantly smaller than the stiffness increment of DC-NPDs (~3%). Therefore, the stiffness increment of DC-NPD specimens is obvious, and such an increment is detectable only with picosecond ultrasound spectroscopy, the most accurate method. Refractive-index measurement The refractive index is needed for calculating the elastic constant from the Brillouin-oscillation frequency. It was measured by ellipsometry [31] using instrument M-2000R produced by J. A. Woollam Co. The ellipsometric angles Ψ and Δ were measured as a function of the wavelength between 380 and 1,700 nm, and the Cauchy model ( n = A 1 + A 2 λ −2 + A 3 λ −4 , where A 1 , A 2 , A 3 are fitting parameters) was used to determine inversely the parameters required for calculating the refractive index. Three independent measurements were conducted for three incident angles of 60°, 70° and 75° for each specimen, and the results were used together in the inverse calculation. Supplementary Fig. S6 shows a typical result for ellipsometry refractive-index measurement. Ab initio calculation of elastic constants The twinned structures in Fig. 3 show transverse isotropy and possess five independent elastic constants, C 11 , C 12 , C 13 , C 33 and C 44 , where the x 3 axis is along the out-of-plane direction. We applied seven deformation modes to the optimized structures with the strain amplitude of 0.01 and calculated energy change. Then, using the harmonic-oscillator approximation, we extracted the second-order elastic constants from the relationships between applied strain and energy increase. The results are shown in Supplementary Table S1 . Supplementary Fig. S2 shows examples of such calculations for the C2-H1 model in Fig. 3c . (For cubic diamond, conversion of the three cubic C ij into the five C ij with (111) transverse-isotropic plane took two steps. First, the cubic C ij were transformed into those in the coordinate system where the x 3 axis was along the [111] direction. Second, thus-obtained C ij was averaged around the x 3 axis by the Hill approximation to yield the average-over- θ C ij [32] .) Compared with lattice parameters, the elastic constants are much more sensitive to interatomic potential, and a larger discrepancy occurs between the ab initio -calculation elastic stiffness with measurement. Even in the calculation of the bulk modulus, for which we expect the highest calculation accuracy because of the simple deformation mode, a 2–3% variation easily appears, depending on the potential as shown in Supplementary Table S2 . We used the pseudopotential given by Rappe et al . [33] , which is based on GGA with the method proposed by Perdew et al . [34] (GGA-PBE). Our bulk moduli are close to those by Wang and Ye [35] when the GGA-PBE potential was used. Predicted elastic-constant increment ( Fig. 4b ) is smaller than observation ( Fig. 2c ). However, such a discrepancy (~3%) occurs often in ab initio calculations, depending on calculation parameters, and especially on the potentials as shown in Supplementary Table S2 . However, the GGA-PBE potential predicts higher bulk modulus of hexagonal phase than that of cubic phase. The point is that our twin-model calculation points in the correct direction and no alternative model is obvious. How to cite this article: Tanigaki, K. et al . Observation of higher stiffness in nanopolycrystal diamond than monocrystal diamond. Nat. Commun. 4:2343 doi: 10.1038/ncomms3343 (2013).